Molecular Russian dolls The host-guest recognition between two macrocycles to form hierarchical non-intertwined ring-in-ring assemblies remains an interesting and challenging target in noncovalent synthesis. Herein, we report the design and characterization of a box-in-box assembly on the basis of host-guest radical-pairing interactions between two rigid diradical dicationic cyclophanes. One striking feature of the box-in-box complex is its ability to host various 1,4-disubstituted benzene derivatives inside as a third component in the cavity of the smaller of the two diradical dicationic cyclophanes to produce hierarchical Russian doll like assemblies. These results highlight the utility of matching the dimensions of two different cyclophanes as an efficient approach for developing new hybrid supramolecular assemblies with radical-paired ring-in-ring complexes and smaller neutral guest molecules. The past five decades have witnessed the rise and flourishing of host–guest and supramolecular chemistry [1] , [2] , [3] , [4] , [5] , [6] , [7] , [8] , [9] , [10] , [11] , [12] . Various macrocyclic hosts have been described in the literature based on diverse noncovalent bonding interactions for recognizing specific guests such as small molecules [13] , ions [14] , biomolecules [15] , fullerenes [16] , and more [17] . The host–guest recognition between two macrocycles to form hierarchical non-intertwined ring-in-ring or host-in-host assemblies, however, remains an interesting and challenging target in noncovalent synthesis [18] , [19] , [20] , [21] , [22] , [23] , [24] , [25] . Such complexes are promising precursors for constructing Russian doll-like superstructures [26] , [27] , [28] , [29] , [30] , [31] or higher order mechanically interlocked molecules, such as molecular Borromean rings [32] , [33] . Tetracationic cyclophanes, formed by linking together two π -electron-deficient dicationic 4,4′-bipyridinium (BIPY 2+ ) units, represent an important class of synthetic hosts on account of their ability to bind electron-rich guests to form 1:1 or 1:2 host–guest complexes [34] . Cyclobis(paraquat- p -phenylene) [35] ( CBPQT 4+ ) is the most intensively explored (Fig. 1 ) among these tetracationic cyclophanes because the 6.8 Å centroid-to-centroid distance [13] between the two BIPY 2+ units of this host which is well-suited for accommodating electron-rich planar aromatic guests such as tetrathiafulvalene [36] (TTF), 1,4-bis[2-(2-hydroxyethoxy)]ethoxylbenzene [37] , and others [38] . The diradical dicationic form— CBPQT 2(+•) —of CBPQT 4+ can also act as a host, encapsulating 1,1′-dialkyl-4,4′-bipyridinium radical cations (BIPY +• ) to form a trisradical tricationic complex [BIPY ⊂ CBPQT] 3(+•) . The binding in these trisradical complexes is relatively strong as a result of homophilic radical-pairing interactions (Fig. 1 ) which represented the first examples of radical–radical interactions between host and guest pairs [39] . Many mechanically interlocked molecules [40] , [41] and redox-switchable molecular machines [42] , [43] have been developed subsequently by employing [BIPY ⊂ CBPQT] 3(+•) as a recognition motif. Fig. 1 Design and structures. a Examples of CBPQT 4+ and CBPQT 2(+•) as hosts. b Proposed superstructures of the tetraradical tetracationic box-in-box complex and Russian doll assemblies Full size image Recently, we have expanded [44] the radical recognition motif to a tetraradical tetracationic host–guest complex in which a square-shaped diradical cyclophane [cyclobis(paraquat-4,4′-biphenylene)] 2(+•) ( SqBox 2(+•) ) encapsulates a cyclobis(paraquat- m -phenylene) ( m -CBPQT 2(+•) ) guest. Recognition between these two diradical dicationic cyclophanes is highly selective, while CBPQT 2(+•) and SqBox 2(+•) exhibit [44] , [45] no binding affinity as a consequence of their mismatched sizes. The m -CBPQT 2(+•) cyclophane is, however, unable to encapsulate any guests on account of the relatively small spacing distance between two BIPY +• units, thus precluding its use in the formation of more sophisticated hierarchical superstructures. Herein, we report the design and synthesis of a rigid tetracationic cyclophane 1 4+ with a centroid-to-centroid distance (Fig. 1 ) between two BIPY 2+ units of 13.1 Å, which, in its diradical dicationic state 1 2(+•) , is ideal for encapsulating CBPQT 2(+•) . The strong radical-pairing interactions between 1 2(+•) and CBPQT 2(+•) has led to the formation of a unique tetraradical tetracationic, box-in-box complex. Interestingly, this box-in-box complex can accommodate small aromatic guest molecules inside the void of the CBPQT 2(+•) component to generate a series of tetraradical tetracationic Russian doll assemblies, both in solution and in the solid state. This kind of complexation is rare in the case of organic compounds [26] , [27] , [28] , [29] , [30] , [31] . Synthesis and structural characterization of 1·4PF 6 The tetracationic cyclophane 1· 4PF 6 was obtained (Fig. 2 ) in 42% yield by the 1:1 cyclization between 2 and 3· 2PF 6 with tetrabutylammonium iodide (TBAI) as a catalyst. 1· 4PF 6 was characterized by 1 H, 13 C, 1 H– 1 H COSY and NOE NMR spectroscopies (Supplementary Figures 1 - 4 ), all of which are in support of the existence of a pure highly symmetrical species in solution. Additional evidence for the formation of 1· 4PF 6 was obtained by high-resolution mass spectrometry (HRMS), which detected the species [ M − PF 6 ] + and [ M − 2PF 6 ] 2+ in the gas phase at m / z = 1152.2163 and 505.1264, respectively. Single crystals were obtained by slow vapor diffusion of i Pr 2 O into a MeCN solution of 1· 4PF 6 during 4 days. The solid-state structure of 1· 4PF 6 , which was determined by single-crystal X-ray diffraction (XRD) analysis, indicates (Fig. 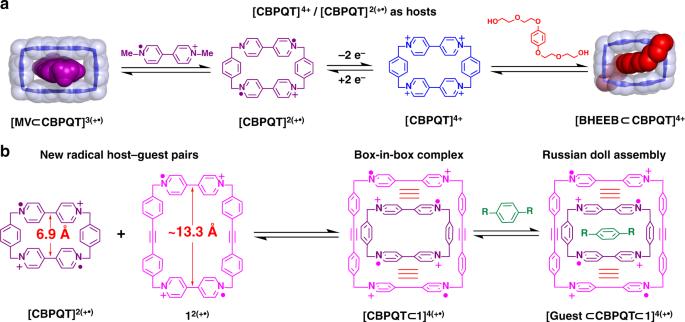Fig. 1 Design and structures.aExamples ofCBPQT4+andCBPQT2(+•)as hosts.bProposed superstructures of the tetraradical tetracationic box-in-box complex and Russian doll assemblies 2 and Supplementary Figure 15 ) that the distance between the two BIPY 2+ units is ca. 13.1 Å. This separation is expected to be ideal for recognition of CBPQT 2(+•) , considering that CBPQT 2(+•) features [46] a 6.9 Å separation of its BIPY +• units, and radical–radical interactions between BIPY +• units typically have spacings [46] , [47] of 3.1–3.3 Å. Fig. 2 Synthesis and crystal structure. a Synthesis of 1· 4PF 6 and b solid-state structure of 1 4+ Full size image Solution phase characterization of the box-in-box complex The association between 1 2(+•) and CBPQT 2(+•) was investigated in the first instance by UV–Vis–NIR spectroscopy. Solutions of 1· 4PF 6 (0.5 mM) and CBPQT· 4PF 6 (0.5 mM) in MeCN were reduced by Zn dust to generate the corresponding radical cyclophanes 1 2(+•) and CBPQT 2(+•) , respectively. Both 1 2(+•) and CBPQT 2(+•) display (Fig. 3a ) very similar absorption bands around 600 nm, an observation which is characteristic of radical cationic BIPY +• absorptions in the absence of radical-pairing interactions. The spectrum of a 1:1 mixture of 1 2(+•) and CBPQT 2(+•) , however, displays an intense new NIR absorption band around 910 nm characteristic [44] , [48] of radical cationic (BIPY +• ) 2 dimers. This observation indicates the formation of a complex between 1 2(+•) and CBPQT 2(+•) as a result of strong radical–radical interactions between the BIPY +• units of 1 2(+•) and CBPQT 2(+•) . In order to estimate the binding affinity between 1 2(+•) and CBPQT 2(+•) , UV–Vis–NIR absorption titrations were carried out by monitoring the change of the NIR absorption band centered on 910 nm. The resulting data could be made to fit a 1:1 isotherm to give (Fig. 3b ) a binding constant of K a = (1.6 ± 0.3) × 10 4 M –1 , which is comparable with that ( K a = 20,000–30,000 M –1 for N -alkyl-substituted BIPY +• ) of [BIPY ⊂ CBPQT] 3(+•) [46] , [47] , and smaller [44] than that ( K a = 1.12 ± 0.08 × 10 5 M –1 ) of [ m -CBPQT ⊂ SqBox] 4(+•) . Fig. 3 UV–Vis–NIR characterization of [ CBPQT ⊂ 1 ] 4(+•) . a UV–Vis–NIR spectra (0.50 mM in MeCN, 1 mm path cuvette) of CBPQT 2(+•) (blue), 1 2(+•) (red), and a 1:1 molar ratio of CBPQT 2(+•) and 1 2(+•) (purple); b Vis/NIR Spectra (MeCN, 2 mm cuvette) on titrating CBPQT 2(+•) into 1 2(•+) (0.10 mM). Initial and final spectra are highlighted in blue and purple, respectively. The inset shows the change in absorption at 910 nm on titration of 1 2(+•) with CBPQT 2(+•) . Curve fitting is highlighted in red Full size image Since the viologen diradical dicationic dimer (BIPY +• ) 2 and the tetraradical tetracationic complex [ m -CBPQT ⊂ SqBox] 4(+•) are reported [44] , [49] to be diamagnetic, based on EPR measurements, the tetraradical tetracationic host–guest complex [ CBPQT ⊂ 1 ] 4(+•) was also expected to be diamagnetic. Thus, we sought to characterize the host–guest complex by 1 H NMR spectroscopy, as we have previously succeeded [45] in doing for the tetraradical tetracationic state of a rotaxane, based on the [ m -CBPQT ⊂ SqBox] 4(+•) recognition motif. At room temperature, however, only a single broad peak near 7.7 ppm was observed in the spectrum (Fig. 4 ) of a 1:1 mixture of 1 2(+•) and CBPQT 2(+•) in CD 3 CN, presumably because of a small thermal population of a paramagnetic state at room temperature [45] , [49] . Upon cooling to –20 °C, the signals of the complex are individually resolved, yet remain broad until further cooling to –40 °C, at which point all of the resonances of the host–guest complex are displayed (Fig. 4 ) as sharp signals. Fig. 4 VT-NMR studies of [ CBPQT ⊂ 1 ] 4(+•) . 1 H NMR Spectra recorded from −40 to +25 °C for a 1:1 molar mixture of CBPQT 2(+•) and 1 2(•+) (1.0 mM each) in CD 3 CN Full size image Since [ CBPQT ⊂ 1 ] 4(+•) is the first radical-pairing-based host–guest complex to be characterized by 1 H NMR spectroscopy, we sought to probe the limits of this technique more deeply for studying supramolecular assemblies featuring radical–radical interactions. Thus, 1 H– 1 H COSY NMR spectra were recorded (Supplementary Figure 6 ) at –40 °C in order to assign the peaks of the host–guest complex. Noticeably, both signals for the aromatic and CH 2 protons on CBPQT 2(+•) are shifted significantly to higher field (Fig. 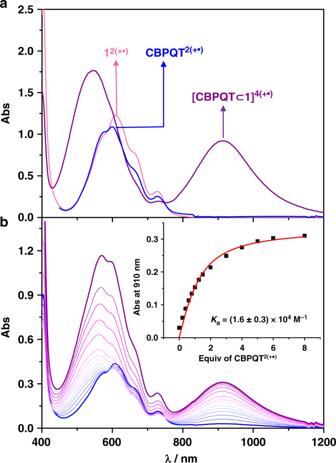Fig. 3 UV–Vis–NIR characterization of [CBPQT⊂1]4(+•).aUV–Vis–NIR spectra (0.50 mM in MeCN, 1 mm path cuvette) ofCBPQT2(+•)(blue),12(+•)(red), and a 1:1 molar ratio ofCBPQT2(+•)and12(+•)(purple);bVis/NIR Spectra (MeCN, 2 mm cuvette) on titratingCBPQT2(+•)into12(•+)(0.10 mM). Initial and final spectra are highlighted in blue and purple, respectively. The inset shows the change in absorption at 910 nm on titration of12(+•)withCBPQT2(+•). Curve fitting is highlighted in red 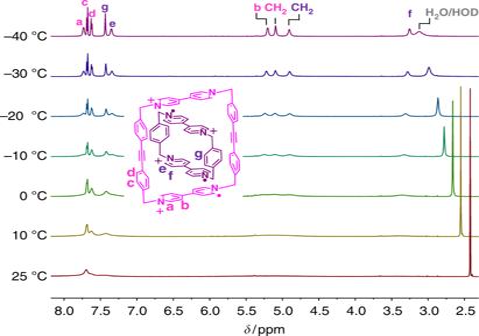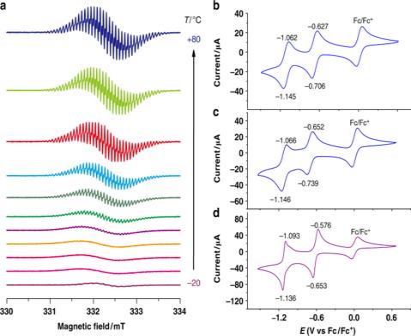Fig. 5 EPR characterization.aEPR Spectra recorded in 10 degree interval on a 1:1 molar mixture ofCBPQT2(+•)and12(+•)(0.50 mM each) in MeCN. Cyclic voltammograms ofb14+(0.20 mM),cCBPQT4+(0.20 mM), andda 1:1 molar mixture of14+andCBPQT4+(0.20 mM each) 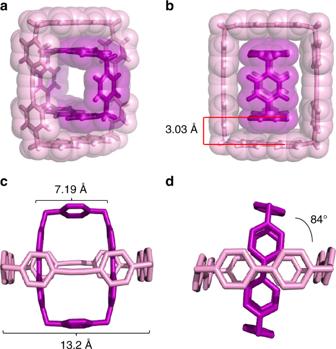Fig. 6 Solid-state superstructures of [CBPQT⊂1]4(+•).aPerspective andbplan views depicted as tubular and space-filling representations.c,dDifferent side-on views, depicted as tubular representations. Hydrogen atoms incanddare omitted for the sake of clarity Fig. 4 VT-NMR studies of [CBPQT⊂1]4(+•).1H NMR Spectra recorded from −40 to +25 °C for a 1:1 molar mixture ofCBPQT2(+•)and12(•+)(1.0 mM each) in CD3CN 4 ) as a consequence of the stronger shielding effect of the host–guest interactions compared with that of 1 2(+•) . Resonances for the meta positions of the pyridinium units in 1 2(+•) and CBPQT 2(+•) which were located at 5.22 (peak b in Fig. 4 ) and 3.28 ppm (peak f in Fig. 4 ), respectively, are shifted to considerably higher fields than those of the ortho protons of the pyridinium units (7.73 ppm for peak a and 7.34 ppm for peak e in Fig. 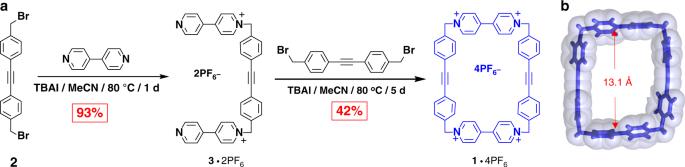4 ). This observation is in line with the solid-state superstructure (Fig. 6 , see below) of the complex [ CBPQT ⊂ 1 ] 4(+•) , which shows that the BIPY +• units in the radical dimers (BIPY +• ) 2 are nearly perpendicular to each other, torsion angle 84°, such that the meta CHs of the BIPY +• units in 1 2(+•) and CBPQT 2(+•) are strongly shielded [45] , while the ortho CHs are not shielded. CW-EPR spectroscopy experiments were carried out in order to probe the electronic structure of [ CBPQT ⊂ 1 ] 4(+•) . Fig. 2 Synthesis and crystal structure.aSynthesis of1·4PF6andbsolid-state structure of14+ The EPR spectrum of CBPQT 2(+•) (298 K, 0.50 mM, Supplementary Figure 22 ) displays almost no hyperfine structure. This observation is a characteristic result of the unpaired electrons in the two BIPY +• units being close enough together for electronic overlap such that spin-exchange interactions between them dominate the spectrum [39] . The EPR (298 K, 0.50 mM, Supplementary Figure 22 ) spectrum of 1 2(+•) exhibits, however, hyperfine splitting which resembles that of other N , N′ -dialkyl substituted BIPY +• radical cations reported in the literature [39] , [46] , since the relatively longer separation distance between two BIPY +• units leads to the absence of efficient overlap for spin-exchange interactions. In comparison, the EPR spectrum (298 K, 0.25 mM each, Supplementary Figure 22 ) of a 1:1 mixture of 1 2(+•) and CBPQT 2(+•) exhibits relatively minimal hyperfine structure. This implies a disruption of the spin-exchange interactions between the two BIPY +• radicals by an interaction (complexation) between 1 2(+•) and CBPQT 2(+•) . Variable-temperature EPR spectra (Fig. 5a ) of the 1:1 mixture of 1 2(+•) and CBPQT 2(+•) in MeCN was then measured at temperatures ranging from –20 to 80 °C. The EPR spectra at −20 °C of the 1:1 mixture displays almost no microwave absorption by unpaired radicals. This indicates that there is strong association of the cyclophanes to form the radical-paired ground state of the complex [ CBPQT ⊂ 1 ] 4(+•) , an observation which is consistent with the VT-NMR results. Upon heating from −20 to 80 °C, the EPR signal of the mixture gradually increased in intensity, along with an increase in the appearance of hyperfine structure. This observation is ascribed to the temperature-induced dissociation of the box-in-box complex into its individual radical cyclophane components. Fig. 5 EPR characterization. a EPR Spectra recorded in 10 degree interval on a 1:1 molar mixture of CBPQT 2(+•) and 1 2(+•) (0.50 mM each) in MeCN. Cyclic voltammograms of b 1 4 + (0.20 mM), c CBPQT 4+ (0.20 mM), and d a 1:1 molar mixture of 1 4 + and CBPQT 4+ (0.20 mM each) Full size image In order to gain insight into the redox processes involved in the assembly and disassembly of [ CBPQT ⊂ 1 ] 4(+•) , cyclic voltammetry (CV) experiments were performed using ferrocene as the internal redox standard. Both CBPQT· 4PF 6 and 1· 4PF 6 (concentration: 0.20 mM in MeCN containing 0.1 M NBu 4 PF 6 , scan rate: 0.2 V/s) exhibit (Fig. 5b, c ) similar reversible redox waves, though the waves for CBPQT· 4PF 6 are more positively shifted than those of 1· 4PF 6 , presumably because of its higher ring strain, resulting from the smaller ring size. CVs of an equimolar mixture of CBPQT· 4PF 6 and 1· 4PF 6 were also measured (Fig. 5d ) at a concentration of 0.20 mM for each box. With a scan rate of 0.2 V/s, the equimolar mixture displays two sharp reversible redox waves, similar to those of the individual boxes, but shifted to more positive potentials. The shifts in the potentials of the redox waves for the mixture of CBPQT· 4PF 6 and 1· 4PF 6 can be rationalized by the formation of a tetraradical tetracationic host–guest complex since radical-pairing interactions will lend stability to the radical cationic redox states, as observed previously [39] , [46] for other radical-based host–guest complexes. Furthermore, CV experiments which were carried out at different scan rates show scan rate-dependent CV behavior (Supplementary Figure 14 ) similar [46] to that of the [ BIPY ⊂ CBPQT ] 3(+•) complex. Solid-state structure of the box-in-box complex Single crystals of [CBPQT ⊂ 1 ]•4PF 6 were obtained by vapor diffusion of i Pr 2 O at room temperature under an atmosphere of N 2 into a solution of an equimolar mixture of 1 •4PF 6 and CBPQT •4PF 6 which had been reduced over Zn dust in MeCN and filtered. Single-crystal X-ray diffraction analysis revealed (Fig. 6 , Supplementary Figure 16 ) a solid-state superstructure in which CBPQT 2(+•) is encapsulated inside the cavity of the 1 2(+•) ring to form a 1:1 host–guest inclusion complex that is consistent with the results found in solution. Fig. 6 Solid-state superstructures of [ CBPQT ⊂ 1 ] 4(+•) . a Perspective and b plan views depicted as tubular and space-filling representations. c , d Different side-on views, depicted as tubular representations. Hydrogen atoms in c and d are omitted for the sake of clarity Full size image The CBPQT 2(+•) ring in the [ CBPQT ⊂ 1 ] 4(+•) complex has a larger BIPY +• centroid-to-centroid distance (7.19 Å) than that [49] observed (6.92 Å) in the solid-state structure of CBPQT· 2PF 6 . The BIPY +• centroid-to-centroid distance is 13.2 Å for 1 2(+•) in the [ CBPQT ⊂ 1 ] 4(+•) complex (Fig. 6c ), which is similar to that (13.1 Å) obtained for 1· 4PF 6 . This observation indicates that the CBPQT 2(+•) ring has to expand slightly in order to optimize binding of 1 2(+•) in its cavity. The torsional angle between BIPY (+•) units of 1 2(•+) and CBPQT 2(+•) is about 84° (Fig. 6d ), which is an energetically favorable angle for BIPY •+ radical pimers, according to theoretical predictions [48] . It is noteworthy that the centroid-to-centroid distance between the adjacent viologen units of 1 2(+•) and CBPQT 2(+•) is only 3.03 Å (Fig. 6a, b ), which is shorter than the spacings (3.1–3.3 Å) that are usually observed [44] , [46] , [47] for viologen radical-pairing interactions. This distance indicates the presence of strong radical-pairing interactions in the solid state, an observation which is consistent with the results of UV–Vis–NIR and 1 H NMR spectroscopic investigations in solution. The extended superstructure reveals (Supplementary Figure 16d ) intermolecular co-facial π-stacking between the radical cationic viologen units of 1 2(+•) , which are similar to that observed [46] , [47] in the solid-state superstructure of [BIPY ⊂ CBPQT] 3(+•) . The centroid-to-centroid separation is 3.48 Å between the co-facially stacked BIPY +• radical cationic subunits of adjacent [ CBPQT ⊂ 1 ] 4(+•) complexes, a distance that is typical for [π···π] interactions, but longer than those (3.1–3.3 Å) typically observed [44] , [46] , [47] for BIPY +• radical-pairing. This observation suggests that the strength of radical-pairing interactions between adjacent complexes might be attenuated since all of the single electrons of the BIPY +• units of 1 2(•+) and CBPQT 2(+•) are strongly paired in interactions that are localized within the [ CBPQT ⊂ 1 ] 4(+•) complex. Formation of Russian doll assembly Notably, the solid-state superstructure of the box-in-box complex [ CBPQT ⊂ 1 ] 4(+•) , confirmed the presence of a void inside of the smaller CBPQT 2(+•) cyclophane component that is large enough to potentially accommodate a second guest. We thus sought out guest molecules that could occupy this cavity to form a Russian doll-like assembly. Radical cationic dimethyl viologen ( MV +• ) was firstly employed as the guest in order to investigate the possibility of forming a pentaradical pentacationic [ MV ⊂ CBPQT ⊂ 1 ] 5(+•) complex. Neither UV–Vis–NIR spectroscopy nor X-ray crystallography, however, indicated the formation of this three-component assembly. We attribute this observation to the limited space between the p -phenylene and bis( p -phenylene)ethyne spacers of the two cyclophanes in [ CBPQT ⊂ 1 ] 4(+•) , which might not provide a large enough window for MV +• to thread. Smaller neutral guest molecules, such as 1,4-dichlorobenzene, were employed in an effort to find guests that could fit into the cavity of the [ CBPQT ⊂ 1 ] 4(+•) complex. These investigations were facilitated by the ability to observe well-defined 1 H NMR spectra of [ CBPQT ⊂ 1 ] 4(+•) at reduced temperatures, and thus, 1 equiv 1,4-dichlorobenzene was added to a 1.0 mM solution of [ CBPQT ⊂ 1 ] 4(+•) in CD 3 CN, and VT 1 H NMR spectra were recorded. Upon decreasing the temperature from 25 to −40 °C, the signals (Fig. 7 ) of a three-component [ p -C 6 H 4 Cl 2 ⊂ CBPQT ⊂ 1] 4(+•) complex gradually appeared and sharpened into well-resolved signals. The formation of the three-component complex was evident from the change in the chemical shifts of all the peaks of the two cyclophane components from those that were observed (Fig. 4 ) for the two component complex [ CBPQT ⊂ 1 ] 4(+•) in the absence of 1,4-dichlorobenzene. The signals of the BIPY +• units, in particular, were shifted significantly to higher fields. The encapsulating of 1,4-dichlorobenzene was further confirmed by the observation (Fig. 7 ) of a new singlet resonance for this guest near 4 ppm. 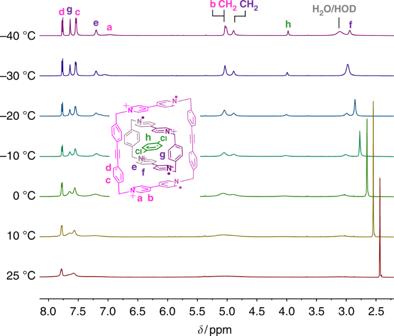Fig. 7 VT-NMR studies of [p-C6H4Cl2⊂CBPQT⊂1]4(+•) 1H NMR Spectra recorded from −40 to +25 °C for a 1:1:1 molar mixture ofCBPQT2(+•),12(+•)and 1,4-dichlorobenzene (1.0 mM each) in CD3CN 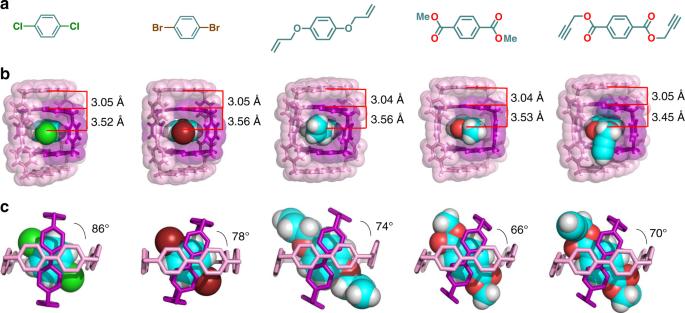Fig. 8 Solid-state superstructure of Russian doll assemblies with different guests inside the [CBPQT⊂1]4(+•)complex.aStructural formulas of the guest molecules.bPerspective views depicted as tubular and space-filling representations.cSide-on views depicted as tubular representations. Hydrogen atoms are omitted for the sake of clarity All these observations indicated that 1,4-dichlorobenzene was encapsulated by [ CBPQT ⊂ 1 ] 4(+•) in CD 3 CN solution, leading to upfield chemical shifts of the signals of the cyclophane components of the complex and to ca. 4 ppm for the 1,4-dichlorobenzene guest that is surrounded on both sides by the CBPQT 2(+•) component of the three-component [ p -C 6 H 4 Cl 2 ⊂ CBPQT ⊂ 1] 4(+•) complex. Fig. 7 VT-NMR studies of [ p -C 6 H 4 Cl 2 ⊂ CBPQT ⊂ 1 ] 4(+•) 1 H NMR Spectra recorded from −40 to +25 °C for a 1:1:1 molar mixture of CBPQT 2(+•) , 1 2(+•) and 1,4-dichlorobenzene (1.0 mM each) in CD 3 CN Full size image One matter that is worth investigating is whether the inclusion of the third component guest ( p -C 6 H 4 Cl 2 ) will affect the binding affinity between CBPQT 2(+•) and 1 2(+•) . Thus, we repeated the UV–Vis–NIR titration experiments with p -C 6 H 4 Cl 2 presented in the solution. By titrating CBPQT 2(+•) into the solution mixture of 1 2(+•) and a number of equivalents of p -C 6 H 4 Cl 2 , similar 1:1 fitting isotherms can be applied to the titration data, and “apparent” binding constants were obtained. Notably, the existence of p -C 6 H 4 Cl 2 guests did, indeed, increase the binding affinity between 1 2(+•) and CBPQT 2(+•) ; the more equivalents of p -C 6 H 4 Cl 2 that were added, the more the binding affinity increased. For instance, when 2.0 eq. p -C 6 H 4 Cl 2 was present, the “apparent” binding constant was found to be (3.8 ± 0.3) × 10 4 M –1 (Supplementary Figure 11 ), which is 1.3 times higher than that of the box-in-box complex without p -C 6 H 4 Cl 2 ; and when the equivalents of p -C 6 H 4 Cl 2 were 6.7 and 20, the “apparent” binding constant increased to (6.2 ± 0.7) × 10 4 M –1 (Supplementary Figure 12 ) and (9.0 ± 1.2) × 10 4 M –1 (Supplementary Figure 13 ), respectively. These results demonstrate that the inclusion of p -C 6 H 4 Cl 2 within the cavity of [ CBPQT ⊂ 1 ] 4(+•) can help to stabilize the box-in-box assembled complex and enhance the binding affinity of [ CBPQT ⊂ 1 ] 4(+•) . The formation of a three-component inclusion complex was confirmed in the solid-state by single-crystal XRD characterization of the superstructure of [ p -C 6 H 4 Cl 2 ⊂ CBPQT ⊂ 1] •4PF 6 . Single crystals of this assembly were obtained by slow vapor diffusion of i Pr 2 O into a mixture of 1 equiv of [ CBPQT ⊂ 1 ] 4(+•) and 4 equiv of 1,4-dichlorobenzene in MeCN. The superstructure shows (Fig. 8 and Supplementary Figure 16 ) that 1,4-dichlorobenzene molecule is located inside the cavity of the [ CBPQT ⊂ 1 ] 4(+•) complex to form the desired Russian doll-like [ p -C 6 H 4 Cl 2 ⊂ CBPQT ⊂ 1 ] 4(+•) complex. The co-conformation of the two cyclophane components within the three-component complex remains almost the same (Fig. 6 ) as in the complex [ CBPQT ⊂ 1 ] 4(+•) in the absence of an additional guest, with the three-component complex exhibiting a contact distance between BIPY •+ units of 3.05 Å and a torsion angle of 86°. The distance between 1,4-dichlorobenzene and the adjacent BIPY •+ units is 3.55 Å, an observation that indicates the presence of [ π ··· π ] interactions between 1,4-dichlorobenzene and CBPQT 2(+•) . The two Cl atoms of the guest are located at the “windows” between the two cyclophanes and exhibit short Cl···H contact distances (2.97 and 3.03 Å) with the two ortho H-atoms of the bis(phenylene)ethyne units. This observation indicates the existence of weak [C–H···Cl] hydrogen bonds between the diphenylethyne units and dichlorobenzene guest, which providing additional stabilization of the Russian doll assembly. The successful formation of a three-component complex with 1,4-dichlorobenzene prompted us to explore other 1,4-substituted benzene derivatives—namely, 1,4-dibromobenzene, dimethyl terephthalate, 1,4-bis(allyloxy)benzene and bis(propargyl)-terephthalate—as guest molecules to bind inside the [ CBPQT ⊂ 1 ] 4(+•) complex. All these molecules were found to form Russian doll assemblies (Fig. 8 , Supplementary Figure 17-21 ) in the solid-state that are similar to the three-component complex formed with 1,4-dichlorobenzene. The contact distances between the BIPY +• units of two cyclophane components are nearly identical (3.04–3.05 Å, Fig. 8 ) for all of the Russian doll assemblies. The torsion angles, however, vary significantly for different guest molecules—86° for 1,4-dichlorobenzene, 78° for 1,4-dibromobenzene, 74° for 1,4-bis(allyloxy)benzene, 70° for 1,4-bis(propargyl)-terephthalate and 66° for dimethyl terephthalate—reflecting the steric influence of the 1,4-substituents on these benzene derivatives. In addition, the accommodation of different guest molecules significantly influences the packing properties (Supplementary Figure 17-21 ) of the complexes. It is noteworthy that [ 1,4-bis(allyloxy)benzene ⊂ CBPQT ⊂ 1 ] 4(+•) and [ 1,4-bis(propargyl)-terephthalate ⊂ CBPQT ⊂ 1 ] 4(+•) are ring-in-ring-type pseudo[3]rotaxanes with vinyl or alkynyl functional groups at the end of the dumbbells, making these assemblies potential precursors for preparing new mechanically interlocked molecules [45] , [50] and redox-controlled molecular machines [51] . Fig. 8 Solid-state superstructure of Russian doll assemblies with different guests inside the [ CBPQT ⊂ 1 ] 4(+•) complex. a Structural formulas of the guest molecules. b Perspective views depicted as tubular and space-filling representations. c Side-on views depicted as tubular representations. Hydrogen atoms are omitted for the sake of clarity Full size image As detailed above, we have synthesized a tetracationic cyclophane that was designed to act as a size-complementary host for recognizing the smaller CBPQT 4+ cyclophane upon reduction of both cyclophanes to their diradical dicationic states. Radical-pairing interactions between the two cyclophanes drives the formation of a novel tetraradical tetracationic box-in-box complex [ CBPQT ⊂ 1 ] 4(+•) , which was investigated thoroughly in solution by spectroscopic techniques (UV–Vis–NIR, VT-EPR, VT- 1 H-NMR) and cyclic voltammetry. An association constant of K a = (1.6 ± 0.2) × 10 4 M –1 was determined on the basis of UV–Vis–NIR titration experiments, and EPR measurements confirmed strong radical-pairing between the cyclophanes to produce a diamagnetic assembly. Remarkably, the radical-pairing interactions are strong enough to permit characterization of [ CBPQT ⊂ 1 ] 4(+•) by 1 H NMR spectroscopy—the first time this technique has been used for characterizing a supramolecular assembly held together by radical–radical interactions. Characterization by 1 H NMR spectroscopy provided detailed information about the co-conformation of [ CBPQT ⊂ 1 ] 4(+•) in solution, which was consistent with the solid-state superstructure that was determined by single-crystal XRD analysis. The most notable feature of the box-in-box complex is its ability to bind various 1,4-disubstituted benzene derivatives inside the cavity of the smaller cyclophane to form hierarchical Russian doll assemblies, which is quite rare in supramolecular systems. Besides, the inclusion of third component guests within the cavity of the box-in-box complex can help to stabilize the assembled structures. These three-component assemblies were characterized in the solid-state by single-crystal XRD analysis, as well as in solution by 1 H NMR spectroscopy. The formation of these hierarchical complexes highlights the box-in-box complex as an attractive motif for forming sophisticated supramolecular assemblies that could be used for designing complicated new mechanically interlocked structures and redox-controllable molecular machines. Thus, this research demonstrates the utility of precisely designing the dimensions of a host for binding a specific guest, such as a smaller cyclophane, that imbues the resulting host–guest complex with appealing properties and functionalities. Materials Solvents used in experiments involving radicals were degassed using the freeze-pump-thaw method. The tetracationic cyclobis(paraquat- p -phenylene) tetrakis(hexafluorophosphate) ( CBPQT •4PF 6 ) was prepared according to literature procedures. Synthesis of 3•2PF 6 4,4′-Bipyridine (4.0 g, 25.6 mmol) was dissolved in MeCN (60 mL), and the solution was heated to 90 °C. Compound 2 (1.3 g, 4.12 mmol) was added in three portions within 1 h. The solution was cooled to room temperature after refluxing for 24 h, and then TBACl (2.5 g, 9.0 mmol) was added. The precipitate was collected by filtration, washed twice with MeCN, and then dissolved in H 2 O. Excess of NH 4 PF 6 was added to the aqueous solution, and the precipitate was collected by filtration and washed successively with H 2 O, MeOH, and Et 2 O. After drying in air, 3 •2PF 6 was obtained as white solid (3.09 g, 93%). 1 H NMR (500 MHz, CD 3 CN) δ 8.47‒8.30, (m, 8 H), 8.32 (d, J = 6.95 Hz, 4 H), 7.79 (d, J = 6.25 Hz, 4 H), 7.65 (d, J = 8.3 Hz, 4 H), 7.50 (d, J = 8.2 Hz). 13 C NMR (125 MHz, CD 3 CN) δ 150.5, 146.0, 134.9, 133.1, 130.0, 128.2, 124.8, 90.6, 65.2. Synthesis of 1•4PF 6 3 •2PF 6 (806 mg, 1.0 mmol), 2 (380 mg, 1.1 mmol) and TBAI (75 mg, 0.20 mmol) were dissolved in MeCN (600 mL), the solution was then heated to 90 °C and stirred for 5 days. The solution was cooled to room temperature, and TBACl (0.83 g, 3.0 mmol) was added to precipitate the solids. The precipitate was collected by filtration, washed twice with MeCN, and then dissolved in H 2 O. Excess of NH 4 PF 6 was added to the aqueous solution, the precipitate was collected by filtration and washed successively with H 2 O and MeOH. The crude product was purified by column chromatography (SiO 2 : 2% NH 4 PF 6 in Me 2 CO) to afford 1 •4PF 6 as a yellow solid (525 mg, 42%). 1 H NMR (500 MHz, CD 3 CN) δ 8.99 (d, J = 7.0 Hz, 4 H), 8.32 (d, J = 7.0 Hz, 8 H), 8.98 (d, J = 7.0 Hz, 8 H), 7.55 (dd, J = 8.1 Hz, 12.6 Hz, 16 H), 5.81 (s, 8 H). 13 C NMR (126 MHz, CD 3 CN) δ 150.5, 146.0, 134.9, 133.1, 130.0, 128.2, 124.8, 90.6, 65.2. (HRMS-ESI). For 1 •4PF 6 , Calcd for C 52 H 40 F 24 N 4 P 4 : m / z = 1155.2178 [ M –PF 6 ] + , 505.1264 [ M –2PF 6 ] 2+ ; found: 1155.2163 [ M –PF 6 ] + , 505.1264 [ M –2PF 6 ] 2+ . UV–Vis-NIR titration Stock solutions of the fully oxidized viologen derivatives CBPQT• 4PF 6 , 1• 4PF 6 were prepared in an N 2 glovebox. The stock solutions were reduced over activated Zn dust for 10‒15 min with stirring and then filtered to provide deep blue solutions of CBPQT 2(+•) or 1 2(+•) . Syringes were employed to measure and dilute the radical stock solutions to the desired concentrations prior to measurements. Spectra were recorded from 1300 to 400 nm in a sealed 2 mm path length cells during titrating CBPQT 2(+•) (0 to 10 equiv) into 1 2(+•) . Binding constant was obtained by fitting fit a 1:1 isotherm according to literature [47] . EPR measurement Solutions of CBPQT 2(+•) and 1 2(+•) were prepared in N 2 glovebox in the same way as was described for preparing the samples utilized for UV–Vis–NIR measurements. After mixing and/or diluting the radical samples to the desired concentration, 100 μL of each sample was transferred to a quartz EPR tube by syringe. The tubes were sealed with UV-cure resin under an N 2 atmosphere. Cyclic voltammetry measurement Samples for cyclic voltammetry were prepared using an electrolyte solution of 0.1 M Bu 4 NPF 6 in MeCN that was sparged with Ar to remove O 2 . The cyclic voltammograms presented in the main text of the manuscript were recorded under Ar or N 2 using a glassy carbon working electrode, a Pt wire or Pt mesh counter electrode, a silver wire quasi-reference electrode, and an internal standard of ferrocene. VT-NMR measurement The sample solutions were prepared in N 2 glovebox with a similar procedure as described for preparing the samples utilized for UV–Vis–NIR measurements. Variable-temperature 1 H NMR spectra and low temperature 1 H- 1 H COSY NMR were recorded using an Agilent DD2 spectrometer with a 600 MHz working frequency for 1 H nuclei. Crystallizations and X-ray analyses for all complexes For 1• 4PF 6 : Single crystals were grown on the bench-top by slow vapor diffusion of i Pr 2 O into a 1.0 mM solution of 1• 4PF 6 in MeCN over the course of a week. For [CBPQT ⊂ 1] •4PF 6 and all the five Russian doll assemblies: Excess of activated Zn dust was added to a mixture of CBPQT •4PF 6 (1.1 mg, 1.0 µmol), 1 •4PF 6 (1.3 mg, 1.0 µmol) together without additional guests ( [CBPQT ⊂ 1]• 4PF 6 ) or with 4 equiv of the corresponding 1,4-disubstituted benzene derivatives in an N 2 glovebox, and the mixtures were stirred for 20 min. After filtering, the purple solutions were kept under an atmosphere of i Pr 2 O at room temperature for a week to allow slow vapor diffusion to occur. The crystals, which appeared in the tubes, were selected and mounted using oil (Infineum V8512) on a glass fiber and transferred to the cold gas stream cooled by liquid N 2 on Bruker APEX-II CCDs with MX optics Mo-K α or Cu-K α radiation. The structures were solved by direct methods and refined subsequently using OLEX2 software. CCDC 1851540–185146 contain the supplementary crystallographic data for this article. These data can be obtained free of charge from the Cambridge Crystallographic Data Centre via www.ccdc.cam.ac.uk/data_request/cif .